Integrating the biophysical and molecular mechanisms of auditory hair cell mechanotransduction Mechanosensation is a property of all cells. Specialized mechanoreceptor cells augment mechanosensation using organelles that respond across a wide range of stimulus frequencies and intensities. Although mechanosensation is critical for regulating such processes as blood pressure, bladder filling, touch sensation, auditory and vestibular function, molecular mechanisms remain elusive. The best studied systems, Caenorhabditis elegans touch receptors and bacterial mechano-gated ion channels, have the advantage of ease of access, genetic tractability and abundance of material, yet fundamental questions as to modes of force translation remain [1] . Inner ear investigations suffer from a dearth of material, genetic intractability and limited access. Despite these limitations, the past decade has progressed in identifying molecular components of the hair cell mechanotransduction (MET) cascade [2] . Incorporating these new data into existing MET models is a great challenge and is in part an aim of this review. The goal of the present review is to provide insight into the mechanisms of MET by integrating biophysical data with genetic, molecular, developmental and immunohistochemical findings, pointing out where long-standing theories need revising and where future work needs to focus. Airborne vibration enters the external ear canal, where it is converted to mechanical vibration by the highly specialized middle ear. The middle ear contacts the cochlea end organ via the stapes bone coupling to the round window. Here vibration is converted into a pressure wave that extends throughout the inner ear and cochlea. In the cochlea, the complex pressure wave is separated into frequency components that vibrate the basilar membrane in a tonotopic manner, with low frequencies represented at the apex and high frequencies at the base. Basilar membrane vibration stimulates the sensory hair cell by creating a shearing force in a specialized organelle, the hair bundle, due to its coupling to a more rigid tectorial membrane ( Fig. 1 ). 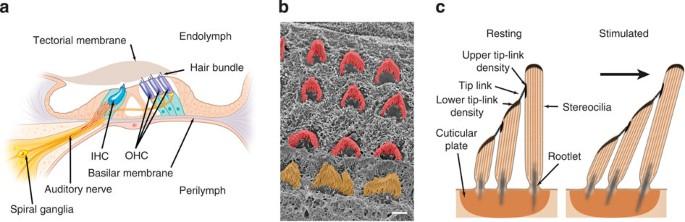Figure 1: Introduction to the organ of Corti. (a) Cross-section of the organ of Corti pointing out the salient features relevant to hearing transduction. Hair bundles on the apical surface of inner hair cells (IHCs) and outer hair cells (OHCs) are bathed in endolymph, whereas the basolateral side of hair cells is bathed in perilymph. (b) Scanning electron microscopy image looking at the apical surface of hair cells with the tectorial membrane removed. IHC and OHC hair bundles are pseudo-coloured orange and red, respectively. Scale bar, 2 μm. (c) Enlargment of a schematic of the hair bundle and hair cell apical surface seen ina. Salient features of stereocilia rows that comprise the hair bundle are indicated. When hair bundles are stimulated, the stereocilia are sheared towards the tallest row of stereocilia, this is also defined as the positive direction of stimulation. Figure 1: Introduction to the organ of Corti. ( a ) Cross-section of the organ of Corti pointing out the salient features relevant to hearing transduction. Hair bundles on the apical surface of inner hair cells (IHCs) and outer hair cells (OHCs) are bathed in endolymph, whereas the basolateral side of hair cells is bathed in perilymph. ( b ) Scanning electron microscopy image looking at the apical surface of hair cells with the tectorial membrane removed. IHC and OHC hair bundles are pseudo-coloured orange and red, respectively. Scale bar, 2 μm. ( c ) Enlargment of a schematic of the hair bundle and hair cell apical surface seen in a . Salient features of stereocilia rows that comprise the hair bundle are indicated. When hair bundles are stimulated, the stereocilia are sheared towards the tallest row of stereocilia, this is also defined as the positive direction of stimulation. Full size image Located on the apical surface of sensory hair cells, hair bundles come in different sizes and shapes, varying with species, sensory organelle and hair cell type ( Fig. 2 ) [3] . The hair bundle is critical for establishing the exquisite sensitivity and dynamic range observed in the auditory and vestibular systems [3] . In common to all hair bundles is a stair-cased pattern of actin-filled microvilli (popularly termed stereocilia) increasing in height towards a tall edge ( Fig. 2 ), in some cases with a true cilium, the kinocilium. Hair bundle deflection towards its tall edge opens mechanically gated ion channels, while deflection away from this edge closes channels [3] . Sensitivity to deflection varies with the angle between stimulus direction and the short to tall stereocilia hair bundle axis [4] . Bundle deflection towards the tall edge exerts a force onto a thin filamentous link (tip link) that attaches the top of the shorter stereocilia with the side of the next tallest row ( Figs 1c and 2 ). Tip link orientation provides directional sensitivity [5] . Cadherin 23 (CDH23) and protocadherin 15 (PCDH15) comprise the tip links, with their cytoplasmic domains localizing at the upper and lower tip-link densities, respectively [6] . These molecules also comprise the lateral connectors of developing hair bundles [7] . Force translates from the tip link to a mechanically gated channel located near the stereocilia tops in proximity to PCDH15 ( Fig. 2 , red and orange stereocilia are predicted to have mechanosensitive channels) [8] . The tip-link requirement for MET is supported by MET loss correlating with tip-link loss, reappearance of tip links correlating with MET return and selective interference of tip-link components inhibiting MET recovery [9] , [10] , [11] . 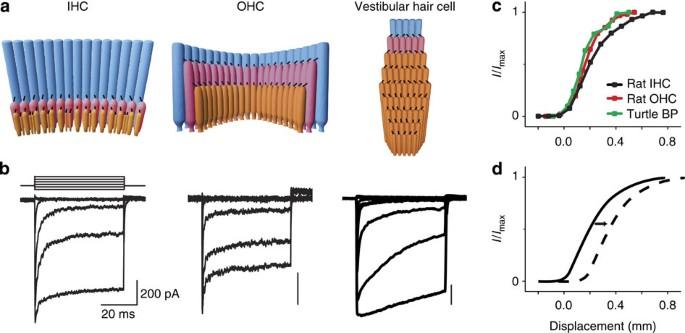Figure 2: Hair bundles and MET vary between hair bundle types. (a) Three distinct hair bundle morphologies are presented (more subtle variations exist). Some stereocilia (blue) do not have functional mechanotransducer channels, whereas others (pink) have functional channels but no direct means of regulating slow adaptation. Orange stereocilia have both functional channels and can be indirectly modulated by slow adaptation. IHC, inner hair cell; OHC, outer hair cell. (b) A family of MET currents from an inner, outer and turtle auditory hair cell are shown, where the cells were voltage clamped at −84 mV and the hair bundles deflected with a stiff rod between −200 and 800 nm (scale bars are the same in all panels). Both fast and slow adaptations are faster in mammalian hair cells, while the slow component of adaptation is more prominent in the turtle (multi-rowed) hair bundle. (c) Plots the current-displacement function for the data inbshowing that IHCs are less sensitive than other hair bundles. (d) Adaptation causes a shift in the activation curve as schematically represented here. An activation curve generated about the hair bundle's resting position is depicted as the solid line, and an activation curve taken from a statically displaced hair bundle is depicted as the dashed line, demonstrating the extended dynamic range. BP, basilar papilla. Figure 2: Hair bundles and MET vary between hair bundle types. ( a ) Three distinct hair bundle morphologies are presented (more subtle variations exist). Some stereocilia (blue) do not have functional mechanotransducer channels, whereas others (pink) have functional channels but no direct means of regulating slow adaptation. Orange stereocilia have both functional channels and can be indirectly modulated by slow adaptation. IHC, inner hair cell; OHC, outer hair cell. ( b ) A family of MET currents from an inner, outer and turtle auditory hair cell are shown, where the cells were voltage clamped at −84 mV and the hair bundles deflected with a stiff rod between −200 and 800 nm (scale bars are the same in all panels). Both fast and slow adaptations are faster in mammalian hair cells, while the slow component of adaptation is more prominent in the turtle (multi-rowed) hair bundle. ( c ) Plots the current-displacement function for the data in b showing that IHCs are less sensitive than other hair bundles. ( d ) Adaptation causes a shift in the activation curve as schematically represented here. An activation curve generated about the hair bundle's resting position is depicted as the solid line, and an activation curve taken from a statically displaced hair bundle is depicted as the dashed line, demonstrating the extended dynamic range. BP, basilar papilla. Full size image Mechanically gated channels represent a diverse protein class with many biophysically distinct properties ( Table 1 ). This in part comes from the loose definition of mechanosensitive channels, as many ion channels can respond to mechanical stimulus and the function of these channels varies significantly. The identity of the hair cell MET channel remains elusive. Difficulties are largely technical in that there are few channels per hair cell and few hair cells per organ. Despite not having the protein in hand, a great deal of information exists regarding MET channel biophysical properties ( Box 1 ). Separating intrinsic channel properties from those imparted by the complex network of hair bundle proteins is difficult, at present pore properties are considered intrinsic ( Box 1 ); however, voltage-gated channel properties can be altered by accessory proteins and this type of alteration might confound MET channel characterization [12] . Matching the intrinsic native channel properties with those of potential candidate channels is critical for assessing the potential of any channel or subunit combination. To date, native channel properties do not match any known mechanosensitive channel ( Table 1 ). Although transient receptor potential channels (TRPs) are implicated in Drosophila and zebrafish, no mammalian homologues of NompC and TRPN1, respectively, have been identified [13] , [14] , [15] . Known biophysical properties of homomeric TRPs do not match those of the MET channel; however, variations in the single channel properties of the native hair cell MET channel implicate a heteromeric channel [16] . The pharmacology of the native channel is not selective to any specific family of channels [17] ( Table 1 ). Thus, identification of the MET channel remains elusive with no clear preference for channel class or type. Table 1 Known mechanosensitive channels. Full size table Box 1: Pore properties of the MET channel. Although the molecular nature of the MET channel remains elusive, a great deal of information exists regarding the biophysical and pharmacological properties of this important channel [95] . Panels a and b provide cross-sectional and top–down views of the MET channel illustrating putative binding sites and topology. MET channels are nonspecific cation channels with a large Ca 2+ permeability [96] . The channel shows minimal rectification, although lowering external Ca 2+ does unmask some inward rectification [59] . The pore shows anomalous mole fraction behaviour where Ca 2+ permeation is regulated by the specific monovalent ion present, such that ions with lower hydration energy (such as K + or Cs + ) enhance Ca 2+ permeation, whereas higher hydration energy molecules (such as Na + and Li + ) reduce Ca 2+ permeation [36] , [97] . Ca 2+ both blocks and permeates the channel leading to the hypothesis that the unusual endolymph solution bathing the sensory hair bundle ( ∼ 20 μM Ca 2+ and 140 mM K + ) serves to maximize both Ca 2+ entry to drive adaptation, while maximizing total current to drive the receptor potential [36] . The block is related to the ability of Ca 2+ to bind within the channel pore at a site near the middle of the electric field (panels a and b ) [98] . A minimal pore diameter of 1.2 nm was estimated using ion substitution experiments, in part explaining the ability of large cations such as FM1-43 and aminoglycosides to permeate the channel (panels a and b ) [17] . These experiments similarly suggested a large external vestibule where the electronegativity within the vestibule could concentrate ions, in part by dehydration, and are consistent with mammalian MET channel sensitivity to ionic strength [59] . Pharmacologically the MET channel is quite ubiquitous with many large positively charged molecules blocking current in an open channel or permeable channel blocker manner [17] . Thus, there are not specific or selective blockers binding the MET channel directly. The one exception to this may be amiloride, a blocker somewhat selective to mechanically gated channels in general [99] , [100] . Single channel measurements from both turtle and mammalian outer hair cells suggest a tonotopic variation in the conductance such that cells responding to higher frequencies have larger conductances (range from 150 to 300 pS) [16] , [59] . Mammalian inner hair cells do not show this tonotopy. The variation in conductance likely suggests that the MET channel is not of a single type but that the channel may be made of heteromeric subunits, have accessory proteins, and/or splice variants of the channel that may vary tonotopically. The molecular and biophysical mechanisms underlying differences in single channel conductance remain to be elucidated. Although a variety of channels have been posited to be the MET channel, no expressed channels have reproduced all of the biophysical and pharmacological properties of the native channel. However, given the likely diversity of channel components, it may be difficult to absolutely identify individual components. Despite the molecular nature of the MET channel remaining unknown, the kinetics of ion channel activation have been measured, leading to hypotheses about how the MET channel is activated. Figure 2b presents hair cell MET current examples for three hair cell types. Responses are fast, with activation kinetics measured or estimated in the microseconds followed by robust adaptation (a decrease in current amplitude during continued stimulation) [18] . Tonotopic variations in activation kinetics have been described in the turtle; however, mammalian kinetics are still too fast to accurately evaluate [18] . Whether kinetic variations are an ion channel property or a hair bundle mechanical property is unclear. Rapid kinetics promoted the idea of direct mechanical channel activation [19] . Prevailing theories suggest that MET channels are tethered to tip links; however, there is no direct evidence to support this argument. At least four possible modes of channel activation exist ( Fig. 3a ): direct tethering to an extracellular protein, an intracellular protein, to both or to neither. In each case, the tip link may be directly involved in MET channel opening or simply a means of tensioning the membrane. Fast kinetics cannot differentiate between these modes. Despite the popularity of tethered channels across the MET field, little data exist to support the hypothesis. 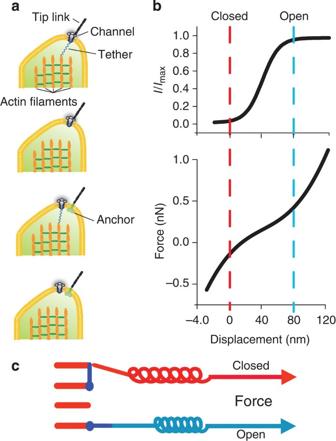Figure 3: Channel gating and the gating spring model. (a) How force is translated to mechanotransducer channels remains to be resolved. At present there are four potential mechanisms, the channel can be tethered (depicted as attached directly to the tip link, although there could be intermediate molecules), internally, externally, both internally and externally, or not tethered at all but simply sensitive to membrane stretch. (b) The upper panel plots the activation curve for the MET channel, whereas the lower panel plots the comparable force-displacement plot. Dashed lines indicate when the channel is fully opened (blue) or fully closed (red). In the force-displacement plot, the reduced slope during the transition from closed to open state in the force-displacement plot underlies the gating spring theory of MET. Depicted incthe gating spring model posits that a gating element moves in series with the spring as the channel opens, thereby reducing tension to the spring transiently, with no required change in spring properties. Figure 3: Channel gating and the gating spring model. ( a ) How force is translated to mechanotransducer channels remains to be resolved. At present there are four potential mechanisms, the channel can be tethered (depicted as attached directly to the tip link, although there could be intermediate molecules), internally, externally, both internally and externally, or not tethered at all but simply sensitive to membrane stretch. ( b ) The upper panel plots the activation curve for the MET channel, whereas the lower panel plots the comparable force-displacement plot. Dashed lines indicate when the channel is fully opened (blue) or fully closed (red). In the force-displacement plot, the reduced slope during the transition from closed to open state in the force-displacement plot underlies the gating spring theory of MET. Depicted in c the gating spring model posits that a gating element moves in series with the spring as the channel opens, thereby reducing tension to the spring transiently, with no required change in spring properties. Full size image Gating spring Unlike a Hookean spring, force applied to the hair bundle produces nonlinear displacement plots with a region of increased compliance correlating with channel gating, the opening and closing of the channel ( Fig. 3b ) [20] . This behaviour underlies the gating spring hypothesis, where a channel gate in series with force application results in increased compliance as the channel activates [20] . The gating spring model suggests a relationship between the force applied to the bundle ( F B ) and hair bundle displacement ( x ): Where K s is the combined stiffness of gating spring and hair bundle pivot, P o is the MET channel open probability, z is the gating force per channel and N is channel number. F 0 is chosen to make F B zero at the hair bundle's resting position. This approach reproduces experimental data well without requiring any specific molecular mechanism to be responsible for the process. Typically for this model type the MET channel is assumed to be a two-state system, with one open and one closed state [20] , [21] , thus Where T is absolute temperature and k is Boltzmann's constant, x 0 is resting bundle position. Figure 3 shows the application of this model, where the two-state Boltzmann plot for channel activation is shown above and the force–displacement plot below. The force–displacement plot shows a nonlinearity during channel activation and linear responses when the channel is either fully opened or fully closed. From this model it is possible to estimate the length of the gating swing, depicted in Figure 3c as the length of the gate that moves in series with the gating spring as the channel opens. Unexpectedly long (9––11 nm) values are obtained, leading to multiple ideas as to the molecular underpinnings of gating swing and spring. Initial hypotheses implicated the tip link; however, structural data and more recent molecular modelling indicate that the tip link is too rigid [22] , [23] . Ankyrin repeats found on some ion channels can create a coiled spring-like structure. These structures are also implicated as potential gating spring components; however, molecular modelling suggest that known repeat motifs would be too stiff [24] . Until the molecular identity of the MET channel is known, this possibility remains viable. One unexplored possibility is lipid stretch. It is possible that distortions in the lipid during bundle deflection lead to nonlinearities of force–displacement plots and that channel gating is simply correlated with this distortion. As more molecules are identified, the likelihood grows that the gating swing reflects a complex molecular interplay and not a simple conformational change in the ion channel ( Fig. 4 ). 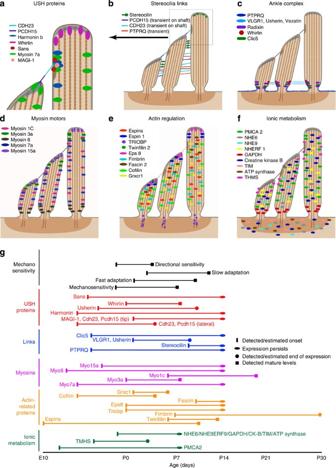Figure 4: Hair bundle proteins. A variety of hair bundle proteins have been identified via genetic and proteomic technologies. These proteins are categorized by general functions into proteins associated with (a) Usher syndrome, (b) stereocilia links, (c) ankle link complex, (d) myosin motors, (e) actin regulation and (f) metabolism and homeostasis. (g) A similar grouping of proteins showing their onset (of detection) and maturation timeline (where applicable) illustrates how the bundle protein composition changes with developmental age. Also included in this timeline plot is the physiological measurements for the onset of MET. Figure 4: Hair bundle proteins. A variety of hair bundle proteins have been identified via genetic and proteomic technologies. These proteins are categorized by general functions into proteins associated with ( a ) Usher syndrome, ( b ) stereocilia links, ( c ) ankle link complex, ( d ) myosin motors, ( e ) actin regulation and ( f ) metabolism and homeostasis. ( g ) A similar grouping of proteins showing their onset (of detection) and maturation timeline (where applicable) illustrates how the bundle protein composition changes with developmental age. Also included in this timeline plot is the physiological measurements for the onset of MET. Full size image Although the gating spring model accurately depicts data obtained, a causal link between channel gating and hair bundle mechanical responses remains to be defined. When first posited, additional hair bundle mechanical components had not been described, in particular adaptation mechanisms were originally thought to have time constants of tens to hundreds of milliseconds. These slower time constants allow for a temporal window, where channels are only activating, so the correlation between mechanics and channel gating appeared strong. However, recent studies show that adaptation is much faster and can be initiated on the submillisecond timescale, thereby shortening the time window separating activation from adaptation ( Fig. 5 ) [18] , [25] , [26] , [27] . Mammalian systems provide clear evidence of the problem ( Fig. 5b ) [28] . Despite these issues, the gating spring model provides an important framework in which to investigate the interplay between hair bundle mechanics and channel gating. 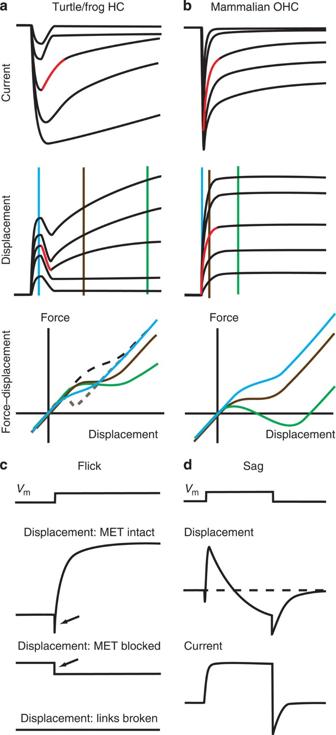Figure 5: Hair bundle mechanics reveal correlations with channel activation and adaptation. (a,b) Upper panels present a schematic of lower frequency (turtle and frog) and higher frequency (mammalian outer hair cell (OHC)) MET currents in response to flexible fibre stimulation. Middle panels present the corresponding hair bundle movements. In each case, the highlighted red curve represents an adaptation response in the current and its correlated movement. These panels further illustrate the correlation between mechanical movement in time and fast adaptation measured in current, suggesting that there is no time point during these measurements where adaptation is not occurring intimating that gating compliance cannot be temporally separated from adaptation. The coloured lines in the middle panel correlate with the lines on the force-displacement plots shown in the bottom panels showing the time course of changes in the force-displacement plots. Similar responses are observed in both high- and low-frequency animals over time, with the main difference between responses being that the mammalian response is much faster, so measurements may be limited by temporal resolution of the recording system. The dashed black line in the force-displacement plot represents an adapted response when compared with the blue line. The dashed grey line depicts negative stiffness, important because it may belie a hair bundle amplification mechanism and also because it challenges whether the gating compliance change is purely a gating phenomenon. (c) Illustrates a voltage-dependent hair bundle movement associated with the MET channel opening (black arrows) that requires functional tip links but not current flow ('the flick'). (d) The currently uncharacterized 'Sag' response is schematized where strong depolarization can move the bundle away from the tall edge and even overshoot the original baseline position (dashed line), without a corresponding reduction in the MET current. This uncoupling of hair bundle position and MET current is unprecedented and may reflect active movements at the cuticular plate. Figure 5: Hair bundle mechanics reveal correlations with channel activation and adaptation. ( a , b ) Upper panels present a schematic of lower frequency (turtle and frog) and higher frequency (mammalian outer hair cell (OHC)) MET currents in response to flexible fibre stimulation. Middle panels present the corresponding hair bundle movements. In each case, the highlighted red curve represents an adaptation response in the current and its correlated movement. These panels further illustrate the correlation between mechanical movement in time and fast adaptation measured in current, suggesting that there is no time point during these measurements where adaptation is not occurring intimating that gating compliance cannot be temporally separated from adaptation. The coloured lines in the middle panel correlate with the lines on the force-displacement plots shown in the bottom panels showing the time course of changes in the force-displacement plots. Similar responses are observed in both high- and low-frequency animals over time, with the main difference between responses being that the mammalian response is much faster, so measurements may be limited by temporal resolution of the recording system. The dashed black line in the force-displacement plot represents an adapted response when compared with the blue line. The dashed grey line depicts negative stiffness, important because it may belie a hair bundle amplification mechanism and also because it challenges whether the gating compliance change is purely a gating phenomenon. ( c ) Illustrates a voltage-dependent hair bundle movement associated with the MET channel opening (black arrows) that requires functional tip links but not current flow ('the flick'). ( d ) The currently uncharacterized 'Sag' response is schematized where strong depolarization can move the bundle away from the tall edge and even overshoot the original baseline position (dashed line), without a corresponding reduction in the MET current. This uncoupling of hair bundle position and MET current is unprecedented and may reflect active movements at the cuticular plate. Full size image A common feature of many mechanoreceptors is adaptation, a reduction in response during a constant stimulus, arising from the receptor's ability to alter its dynamic range. Thus, the decrease in current during a constant stimulation is recovered by further stimulation ( Fig. 2d ) [25] . Adaptation is not unique to hair cells as other mechanically gated ion channels exhibit this phenomenon, namely MEC channels in C. elegans [29] and MscL (mechanosensitive channel of large conductance) channels in bacteria [30] . Whether the molecular mechanisms underlying adaptation are common between mechanoreceptors remains to be determined. Initial investigations of hair cell adaptation suggested a single mechanism, but as will become more evident, at least two independent mechanisms are likely involved. For clarity and historical perspective, common features and possible mechanisms are presented first and then separation of components described. A variety of functions are ascribed to hair cell adaptation. Adaptation shifts the cell's sensitivity range preventing saturation, extending the dynamic range [25] . Where investigated, adaptation functions as a high-pass filter with rates varying with location along the auditory end organ (tonotopically) [18] , [26] , [27] . When coupled with variable activation kinetics, this function creates a band-pass filter to incoming sound, contributing to frequency selectivity [18] . Adaptation serves as an amplifier when coupled with gating compliance [31] . Adaptation provides the resting current (through steady-state MET channel open probability) required to set the hair cell's resting membrane potential [32] , [33] . And finally, adaptation functions as a protective mechanism to hair bundles, limiting damage from large stimulations [25] . Historically, adaptation was considered to be one mechanism driven by Ca 2+ entry through MET channels [25] , [34] , [35] , [36] . Intracellular Ca 2+ buffers alter adaptation suggesting an intracellular effector site for adaptation [26] , [35] . Models of adaptation mechanisms were initially based on hair bundle mechanical measurements; in one case, kinetics were quite fast and no clear mechanical component was identified [34] , [37] . This favoured a channel-based mechanism, where Ca 2+ entry caused a conformational change in the channel, stabilizing a closed state. Little data exist to support or refute this hypothesis; MET channel identification is necessary for direct evaluation. One issue with the channel conformational change model is that activation curves can shift hundreds of nanometres, a range difficult for a channel conformational change to accommodate. A second more accepted adaptation model is based on a measured hair bundle stiffness decrease (relaxation) during adaptation ( Fig. 5 ) [38] . The slow time course of hair bundle relaxation matched the adaptation rate and thus was formed the motor model for adaptation. Here the channel is presumed to be coupled at the upper tip-link insertion point (where the tip link attaches to the membrane in the upper tip-link density). Intracellularly, the channel and link are complexed to myosin and Ca 2+ entry results in the complex releasing from the actin cytoskeleton, slipping down the stereocilia, reducing tension and closing the channel. Channel closure results in reduced stereociliary Ca 2+ allowing myosins to reattach, climb up actin filaments and restore tip-link tension [39] . Over the past 25 years, data supporting the motor model have accumulated. Adaptation requires energy (that is, ATP) [40] . Myosin-Ic is identified at the upper tip-link insertion, localized where expected if climbing and slipping are important (although localization in mammalian outer hair cells is quite variable) [41] , [42] . The tip link is under constant tension supporting a mechanical component to the process [11] . The upper insertion point moves towards the tops of stereocilia upon breakage of the tip link, again supporting a tensioning mechanism [43] . A very clever genetic manipulation of the ATP-binding site of myosin-Ic abolishes adaptation [44] , [45] . The MET channel is localized near stereocilia tops and asserted to be at the upper and lower tip-link density regions, based on indirect Ca 2+ imaging experiments [46] . More recently the myosin-Ic motor model is questioned at multiple levels: distinct adaptation components are described, multiple molecules can alter adaptation properties, developmental onset of adaptation separate from that of myosin-Ic and MET channel localization at stereocilia tips is removed from the site of myosin-Ic. First, data suggest that multiple adaptation components (fast adaptation and slow adaptation) exist and are separable based on kinetics, dynamic range, sensitivity to Ca 2+ , developmental onset and requirement for ATP [18] , [47] , [48] . Fast adaptation (or calcium-dependent channel reclosure) happens on a millisecond (or submillisecond) timescale [27] , [49] , a rate too fast for any conventional myosin motor activity. Fast adaptation rates vary tonotopically in both turtle hair cells and mammalian outer hair cells [18] , whereas slow adaptation rates do not [26] . Fast adaptation is most sensitive about the resting hair bundle position, whereas slow adaptation manifests only with larger stimulations [47] . Fast adaptation is comparable kinetically in responses to both positive and negative hair bundle deflections [47] , whereas slow adaptation is faster for positive stimuli. Fast adaptation appears earlier in development in rat and mouse outer hair cells, whereas slow adaptation appears later [48] , [50] . Fast adaptation is insensitive to ATPase antagonists [47] , whereas slower adaptation requires ATP [40] . Thus, the existence of multiple different forms of adaptation makes it unlikely that a motor model can account for both, especially as fast adaptation rates are too fast. Second, recent experiments question the motor model by implicating the involvement of other proteins that may provide alternative adaptation models. Both myosin-VIIa and myosin-XVa modulate adaptation [51] , [52] . Myosin-XVa does not localize specifically to the upper tip-link densities [53] ; however, animals with non-functioning myosin-XVa have MET currents with no appreciable adaptation response. Recent data suggest that myosin-VIIa may localize near upper insertion points [54] ; however, physiological data suggest adaptation is more robust in animals where myosin-VIIa is non-functional, the major deficit here being a shift to the right of the activation curve [51] . A third molecule, PIP 2 , has a significant role in modifying adaptation, with no clear evidence for how PIP 2 might modulate myosin-Ic. Myosin-Ic can bind and sequester PIP 2 at membranes, and perhaps the role of myosin-Ic is modulatory on PIP 2 (refs 55 , 56 ). These effects demonstrate the complexity of the system where indirect modulation makes it quite difficult to assess causal mechanisms. Third, the myosin-Ic motor model is further challenged by the expression time course and pattern of myosin-Ic. In outer hair cell bundles, myosin-Ic levels peak several days after adaptation has matured [48] , at the very least suggesting another function for the motor not yet determined. And finally, direct imaging of Ca 2+ entry using high-speed confocal microscopy localizes MET channels to stereocilia tips and not at upper tip-link densities where myosin-Ic is localized [8] . Thus, it is unlikely that Ca 2+ entry via MET channels can directly modulate myosin-Ic. Together, a growing body of evidence questions the long-standing myosin motor model and warrants a revamping of the adaptation model. A unifying theory, well grounded in the evidence presented above, suggests the existence of two independent mechanisms present at different stereocilia locations, where one mechanism tightly regulates the fast kinetics of adaptation while the other regulates tip-link tension, and thus the MET channel operating point [57] . In this way motor adaptation tensions tip links to set the operating point, Ca 2+ entering stereocilia through the second row MET channel diffuses to the upper tip-link insertion point, thereby indirectly regulating third row MET channels [58] . Several predictions arise from this theory. First, slow motor adaptation should arise only with larger hair bundle deflections that generate higher stereociliary Ca 2+ concentrations, a property already described (see above). A second prediction is that the extent of adaptation would be greatly reduced in hair bundles with only three rows of stereocilia, given that only about 30% of the stereocilia would be able to adapt at all ( Figure 2a presents potentially adapting stereocilia and non-adapting stereocilia). Inspection of MET currents in Figure 2b supports this possibility, where the slow adaptation is most complete in hair bundles with a larger percentage of adapting stereocilia. This relationship does not correspond to the fast adaptation component. A third prediction is that single channel recordings would not show slow adaptation. Although not explicitly discussed, the ensemble averages are best fit with single exponentials with time constants more in line with fast adaptation [16] , [59] . A third indication that tip-link tension is an indirect effect is that adaptation time constants are slower (at a given tonotopic location) in hair bundles with smaller amplitude MET currents [27] , [57] . Current variations between cells is likely due to mechanical damage during isolation, but the correlation between adaptation rates and MET current amplitudes was previously inexplicable because each stereocilium was considered a unit with a constant Ca 2+ influx, so adaptation at a given position should be constant (that is, there is no summation between stereocilia). In the new hypothesis, loss of some tip links can result in loss of slow adaptation in remaining functional stereocilia and might in part account for the correlation observed (activation would also be predicted to slow due to the loss of tip-link tensioning, thus slowing fast adaptation as well). With this hypothesis, it may be that slow adaptation is a misnomer in that the major function of the indirect effect of the motor system is maintaining tension in the tip link to ensure rapid activation. The adaptive component may only come into action during large stimulations where Ca 2+ can accumulate. This indirect control may also be reflected in the Ca 2+ -dependence of activation [18] . Adaptation may be an independent mechanism more localized to the channel site at the tops of stereocilia. Aside from the adaptation model coming under question, whether slow adaptation is controlled by the same mechanism between hair cell types is also unresolved. Slow adaptation in mammalian auditory hair cells differs from that in vestibular hair cells as well as those from other vertebrates. Adaptation rates are faster in mammalian auditory hair cells ranging from single to tens of milliseconds, whereas in other systems the range is tens to hundreds of milliseconds [25] , [45] , [47] , [48] . Additionally in mammals, myosin-Ic expression lags the onset of slow adaptation, and myosin-Ic is not specifically localized to the upper tip-link densities [48] , [60] . Whether differences between adaptation in different end organs and species are due to differences at the molecular or structural level remain to be determined. The hair bundle does not function as a simple spring with linear movements in response to force stimulation, but rather undergoes stiffness changes correlating with various activation and adaptation components of the MET channels ( Fig. 5 ). The decrease in stiffness correlated with channel opening (gating spring) has already been discussed ( Fig. 3 ). Passive properties Early work demonstrated that stereocilia behave as stiff rods, rotating about their ankles [37] , [61] . Hair bundle deflections cause stereocilia to pivot about the base creating a shearing of adjacent stereocilia. Laser interferometry supports this contention, extending the original work to better demonstrate rigidity and cohesiveness of the bundle [62] . Recent data identified the actin bundling protein TRIOBP as a critical part of the stereocilia rootlet ( Figs 1 and 4e ), decreasing hair bundle compliance by stabilizing this insertion [63] . Specializations in extracellular proteins associated with the stereocilia are postulated to reduce friction between stereocilia enhancing coherent motion [62] . Fast adaptation Hair bundle deflection with a flexible fibre produces a rapid movement in the stimulus direction followed by a rapid rebound against the probe ( Fig. 5a,b ) [38] , [49] , [64] . The rebound time course (negative movement) matches the fast adaptation time course in turtle and frog (see colour coding in Fig. 5a ). The direction of bundle motion can be interpreted in two ways. First, a negative movement with a sustained positive step of the flexible fibre could indicate bundle stiffening during adaptation. Alternatively, it may reflect a shift in the activation curve that moves the nonlinear response component along the displacement axis; therefore, not requiring a stiffness change [49] . Figure 5 presents the shift in the force–displacement plot as a dashed black line. In mammalian outer hair cells, the mechanical response rise time corresponds to fast adaptation (see colour coding in Fig. 5b ) [65] . Whether this reflects a separate mechanism or simply that the stimulus rise time is not fast enough to distinguish activation and adaptation remains to be determined. The original concept for fast adaptation is Ca 2+ entering and binding to a site on the MET channel stabilizing a closed state [20] , [34] , [35] , [65] , [66] . Work with optical trap technology further supports this model, suggesting that a mechanism requiring a hair bundle compliance change is not tenable [64] . Recent data on channel localization would also undermine models involving direct myosin interactions [39] , [67] . Slow adaptation Slow or motor adaptation is the original mode of adaptation described above. The mechanical correlate of slow adaptation is an increase in hair bundle compliance during a force stimulus [38] . Figure 5 depicts the bundle movement and the force–displacement plot. The colour coding for the plots in Figure 5a illustrates how slow adaptation alters the force–displacement relationship in the lower vertebrate organs. The plot showing the time sequence illustrates an increase in breadth of the nonlinear compliant region and a reduction in the slope following full channel activation. Interestingly, a similar plot is found in mammalian hair cells at earlier time points not only suggesting that mammalian measurements were unable to separate mechanical components, but also suggesting similar compliance changes as in lower frequency cells [28] . Responses of mammalian hair cells are considerably faster than responses of turtle/frog hair cells; the main question is whether a similar mechanism can account for the range in kinetic responses between hair bundle types. The interaction of fast and slow adaptation with channel gating compliance can result in a force–displacement plot, where the nonlinear component has a negative slope (dashed grey trace in Fig. 5a ) [31] . This negative stiffness may underlie an active hair bundle amplification process. Negative stiffness may also be seen when looking at hair bundle stiffness at time points when adaptation has a greater contribution to the response (later than stimulus onset; Fig. 5a,b, coloured lines). In this case, turtle/frog hair cell responses at later time points are more similar to their mammalian counterparts at earlier time points. The presence of negative stiffness illustrates the complex interaction between different mechanical components. This raises the question as to whether it is possible to separate gating compliance (see earlier gating spring discussion) from adaptation. Additional hair bundle mechanics Aside from mechanical components associated with either activation or adaptation, several other hair bundle movements are described. A voltage-dependent bundle movement associated with MET channel activation manifests as a step-like movement in both turtle and frog ( Fig. 5c ) [21] , [64] . Termed a 'flick', this movement is independent of current flow through the channel, but is abolished with breaking links using BAPTA. No underlying mechanism for this movement is known. A second movement, termed 'sag', is present in turtle auditory hair cells ( Fig. 5d ) [21] . Here with depolarization, the bundle first moves towards its tall edge while MET channels are opening. Strong depolarizations result in a slow rebound of movement that can overshoot the original baseline position of the hair bundle. This movement is uncoupled from MET current, which remains constant throughout. The sag is slower than adaptation. No underlying mechanism for this movement is available. One interesting possibility is that the sag represents a hair bundle rocking due to cuticular plate curvature changes or rotation so that no change in force at the tip link is observed. In hair bundles attached to a tectorial or otolithic membrane, rocking could result in a closing of MET channels separately from other adaptive processes. And finally, spontaneous bundle oscillations, presenting as either low-frequency limit cycle type behaviour or rapid resonant type behaviour, are described in lower frequency and vestibular hair cells [37] , [68] , [69] . The underlying mechanisms for these movements remain to be identified, as do causal links to the MET channel function. Understanding the steps and time course of development and maturation of MET can provide significant insight into the contributing molecules and mechanisms. Proteins important for the process are predicted to be present at critical time points during development ( Fig. 4g ). Also whether mature MET properties, such as directional sensitivity and adaptation, are inherent in the onset of MET or develop independently over time provides some insight into their mechanisms ( Fig. 6 ). 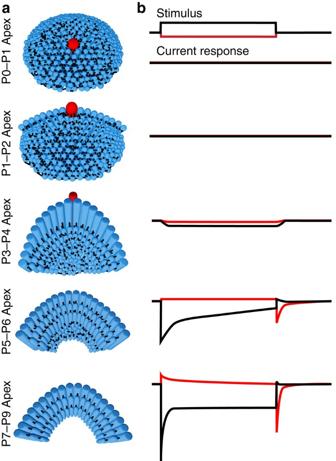Figure 6: Hair bundle and mechanosensitivity develop along similar time frames. (a) Hair bundle development at five distinct stages is illustrated showing how the kinocilium (red), stereocilia (blue) and interciliary links (black) change at each time point. Depicted for apical hair bundles are the tuft stage (P0–P1), the establishment of polarity (P1–P2), the initial height increase (P3–P4), the thickening and pruning (P5–P6) and the final height increase (P7–P9). (b) Corresponding maturation of MET is schematized with responses to negative stimuli away from the tall row (red) and positive towards the tall row to open channels (black). Illustrated are the slow increase in current amplitude, the initial lack of directional sensitivity, and the increase in magnitude and kinetics of adaptation. Figure 6: Hair bundle and mechanosensitivity develop along similar time frames. ( a ) Hair bundle development at five distinct stages is illustrated showing how the kinocilium (red), stereocilia (blue) and interciliary links (black) change at each time point. Depicted for apical hair bundles are the tuft stage (P0–P1), the establishment of polarity (P1–P2), the initial height increase (P3–P4), the thickening and pruning (P5–P6) and the final height increase (P7–P9). ( b ) Corresponding maturation of MET is schematized with responses to negative stimuli away from the tall row (red) and positive towards the tall row to open channels (black). Illustrated are the slow increase in current amplitude, the initial lack of directional sensitivity, and the increase in magnitude and kinetics of adaptation. Full size image Hair bundles begin as patches of short, thin microvilli with a kinocilium [70] in the centre ( Fig. 6a ). The kinocilium migrates to one end of the microvilli patch, while microvilli at that end elongate into stereocilia [71] . The similar directional polarization of all hair bundles is regulated by planar cell polarity proteins, present before bundle formation [72] . Stereocilia grow in length by the addition of actin monomers to the barbed ends of actin filaments at the tips of stereocilia [73] . Following kinocilium migration and initial stereocilia elongation, elongation stops and thickening takes place (in mammals, thickening and elongation overlap temporally [74] ), regulated by bundling proteins such as espins [75] and plastins [71] . Concomitantly, tapering of the stereocilia base occurs, and actin filaments extend into the cuticular plate, forming rootlets [71] . At this point, pruning of additional microvilli begins. The final stage of maturation is a differential increase in stereocilia length, establishing a final staircase pattern, a consistent step regardless of final hair bundle morphology [71] , [74] . Growing evidence suggest that the hair bundle is a dynamic specialization where stereocilia reshaping is an ongoing, energy demanding process [73] . Differences in hair bundle length, thickness, number of stereocilia and staircasing step-size are observed in both auditory and vestibular hair bundles. Molecules and pathways responsible for establishing these important differences remain to be elucidated. As hair bundles mature, interciliary connections remodel and prune ( Figs 4 and 6a ) [76] . There are four distinct linkage types: ankle links, shaft connectors, horizontal top connectors and tip links, described largely by location and less by protein make-up. Ankle links, absent from mature mammalian cells, localize above the tapered base during maturation [76] ; loss of ankle links results in the loss of directional sensitivity, reduced MET and broadened activation curves ( Table 2 ) [77] . The shaft connectors localize to the lower third of avian hair bundles when horizontal top connectors are present, but redistribute along the shaft when top connectors are absent [76] . Top connectors consists of stereocilin that localizes at the tallest row tips of outer hair cells and their respective tectorial membrane imprints [78] . Stereocilin knockout mice have normally developing bundles but fail to maintain their morphology and contact with the tectorial membrane. Progressive hearing loss results from splayed and degenerate bundles [78] . Finally, the tip link, consisting of PCDH15 and cadherin 23, extends obliquely between adjacent rows of stereocilia [5] , [6] . The tip link imparts directional sensitivity to the hair bundle and is required for MET channel activation ( Figs. 1c , 4a ). Table 2 Summary of mouse model phenotypes of hair bundle proteins. Full size table Superimposed onto hair bundle development is the maturation of MET ( Figs 4g and 6b ). In avian [79] and mammalian [48] , [50] , [80] auditory systems, MET matures gradually, where currents are initially small, slow to activate, non-adapting, not directionally sensitive and require large bundle deflections ( Fig. 6b ). Current amplitudes and kinetics mature within 2 days of response onset. Fast adaptation appears within a day of mechanosensitivity and kinetics mature over the next 5 days, correlating with the expression pattern of myosin-IIIa ( Fig. 4g ). The onset of slow adaptation is delayed compared with fast adaptation. The development of slow adaptation precedes and matures faster than the expression of myosin-Ic might predict [48] ( Fig. 4g ). The onset of directional sensitivity corresponds to pruning of interciliary connectors [48] ( Fig. 6 ). Together, these data suggest that proteins are independently transported to stereociliary tips where they are assembled into a functional complex. An alternative hypothesis exists for vestibular hair cells, where data indicate that MET appears immediately mature. 'All or nothing' suggests that the MET complex assembles at the stereocilia base and migrates to the tops, immediately mature and functional [80] . Reconciling these hypotheses is difficult. One possibility is that smaller and less sensitive immature currents are harder to observe in less sensitive vestibular bundles compared with auditory, so in fact maturation would not be different between end organs. New hair bundle proteins are being identified at a rapid rate, with functions still mostly obtuse ( Fig. 4 ). Proteomic and genetic approaches have yielded important findings as to the complexity of hair bundle protein interactions [2] . A major obstacle to ascribing specific protein roles in MET is that many proteins have multiple functions and these functions are closely integrated making it difficult to identify a single causal role for a particular protein. This is most clear in that most animals carrying mutations in genes encoding for hair bundle proteins have severe hair bundle structural deficits onto which MET is imposed ( Table 2 ). Delineating between structural effects and channel activation effects is difficult at best. Adding to the complexity is a common pattern where initial hair bundle phenotypes progress towards a hair bundle loss or resorption and then to hair cell loss, so that causally connecting a protein to even a particular morphology let alone function can be difficult. For simplicity, it is possible to categorize hair bundle proteins into groups, including those associated with Usher syndrome (USH) and stereociliary links, motor proteins, actin regulation, and metabolism and homeostasis. Some of these proteins have already been discussed. Distributions and categories are presented in Figure 4 and Table 2 . Usher syndrome and stereocilia links proteins Human deafness-related mutations shed new light onto hair bundle protein composition, and regulation, in particular those associated with hair bundle links. USH types 1, 2 and 3 are a major cause of deafness–blindness in humans [2] . Type 1, the most severe, involves a variety of mutated molecules associated with the hair bundle, including cadherin-23 (USH1D), protocadherin-15 (USH1F), SANS (USH1G), harmonin (USH1C) and myosin-VIIa (USH1B). In USH type 2, the most frequent, VLGR1 (USH2C), Usherin and whirlin (USH2D) are affected. Mutations leading to USH type 3 involve Clarin-1, a protein thought to be involved in synaptic transmission (USH3A). USH1 proteins are localized to regions of the tip link and tip-link densities. Mutations result in altered shapes, sizes, positioning and overall integrity, features critical for proper MET ( Table 2 ) [81] . Identifying individual protein function as related to MET properties is quite difficult due to the molecular interactions indirectly altering hair bundle mechanics. Motor proteins A variety of unconventional myosin motors are found in stereocilia, showing very distinct localization patterns ( Fig. 4d ; Table 2 ). Functions associated with myosins range from regulating MET adaptation, to transporting hair bundle proteins, to regulation of hair bundle elongation, maintenance and scaffolding. Attributing these functions to the intrinsic ability of the myosin or to the transport of other proteins by myosins has yet to be fully determined. Unconventional myosins-Ic, IIIa, VI, VIIa and XVa are important for hair cell function ( Fig. 4d ). Myosin-Ic is proposed as the motor protein responsible for both fast and slow adaptation (see earlier discussion), but may also serve as a lipid-interacting protein and transporter as in other cell types [82] . Myosin-VIIa interacts with components related to MET machinery, such as scaffolding proteins SANS and harmonin [2] , the tip-link protein protocadherin-15 (ref. 83 ) and the actin-capping factor twinfillin-2 (ref. 84 ), yet where available, the morphological and physiological phenotype of mice carrying mutations in these interacting proteins differ from the myosin-VIIa pheonotype [51] . Myosin-IIIa localizes to stereocilia tips with expression profiles matching that of fast adaptation [48] , [60] . The functional consequence of myosin-IIIa mutations remains to be assessed. Myosin-VI is a minus-end-directed motor, which might function as a transporter of molecules such as PTPRQ [85] , or as an anchoring element [86] between the plasma membrane and the actin core. Myosin-VI knockout mice ( Snell's waltzer ) have profound deafness and loss of balance as early as P1, but functional consequences to MET are yet to be determined. Determining causal links between myosin motor activity and MET function are difficult, with chemical genetic strategy used for myosin-Ic having the strongest data (because there are no developmental anomalies), yet even here, effects on fast adaptation are likely non-causal [44] , [45] . Actin regulation proteins Stereocilia have an actin core structure that is critical for proper MET sensitivity. Stereocilia grow to a specific height and width, both within a given hair bundle and across end organs. Espin and fimbrin [71] , [75] are actin bundlers/crosslinkers in stereocilia, involved in regulating bundle lengthening and thickening. Espins provide the most rigid crosslinking for stereocilia, comprising six different isoforms [87] , where mutations cause cochlear and vestibular dysfunction [75] , [88] in both humans and jerker mice. The Ezrin/Radixin/Moesin group of molecules, known for linking the underlying actin core to the plasma membrane in microvilli [89] , are also expressed within hair bundles. Radixin is expressed in cochlear hair cells, and both radixin and ezrin are expressed in vestibular stereocilia [90] . Actin-capping proteins such as twinfilin and Eps8 are likely also involved in the shaping of stereocilia [84] , [91] , [92] , [93] . Data suggest that stereocilia tops have a beveled shape dictated by the presence of stereociliary links [22] , [73] . The mechanism and time course for reshaping and the molecules that regulate this process are unknown. Presumably, actin treadmilling, where actin monomers are added at the tops of stereocilia and removed at the bottom (at least in neonatal cultured rat hair bundles), underlies much of these actin dynamics [73] . Whether these processes have direct effects on MET on rapid timescales has not yet been investigated. Metabolism and homeostasis proteins Mass spectrometry of hair bundle proteins identified metabolic proteins such as creatine kinase as one of the most abundant in stereocilia ( Fig. 4f ) [94] . This work highlights the dynamic nature of the hair bundle organelle and the large energy demands required for maintenance of proper shape and MET activity. The ability to closely regulate Ca 2+ levels, as well as the various roles of myosins in shaping both stereocilia properties and MET require a high-energy load. Many of these processes are far from a regenerative source of ATP (that is, mitochondria around the cuticular plate) requiring more efficient and rapid supply and storage of energy components, such as the creatine phosphate shuttle. It is possible that many of the pathological conditions such as those related to ototoxicity or noise damage are a reflection of compromised metabolism being unable to maintain hair bundle dynamics. Certainly, a common phenotype under many pathological conditions is the resorption of the hair bundle and then loss of the hair cell. Great strides have been made over the past decade to identify molecular components of the MET process. Although we have come a long way, many of these new findings require a reevaluation of accepted theories. Further investigation is needed to explore the possibility that separate mechanisms exist for maintaining tip-link tension to ensure rapid activation and regulating the MET dynamic range through adaptation. Similarly, the role of the lipid bilayer and the question of whether the MET channel is tethered need more definitive testing. Future experiments need to causally leap between the molecular and cellular, between the morphological and physiological to tease apart specific functions in a complex interwoven network of molecules. To do this, technical advances are also needed. Better resolution, higher speed imaging technologies and faster mechanical fibres need to be applied to the hair bundle. Single cilia physiology is needed to directly test current theories of channel activation and adaptation. Specific means of altering protein function after development are critically important. As transfecting hair cells has had limited success and difficulty with specificity, better means of taking advantage of the molecular and genetic advances at the physiological level are needed. How to cite this article: Peng, A.W. et al . Integrating the biophysical and molecular mechanisms of auditory hair cell mechanotransduction. Nat. Commun. 2:523 doi: 10.1038/ncomms1533 (2011).